Rab6a releases LIS1 from a dynein idling complex and activates dynein for retrograde movement Cytoplasmic dynein drives the movement of a wide range of cargoes towards the minus ends of microtubules. We previously demonstrated that LIS1 forms an idling complex with dynein, which is transported to the plus ends of microtubules by kinesin motors. Here we report that the small GTPase Rab6a is essential for activation of idling dynein. Immunoprecipitation and microtubule pull-down assays reveal that the GTP bound mutant, Rab6a(Q72L), dissociates LIS1 from a LIS1–dynein complex, activating dynein movement in in vitro microtubule gliding assays. We monitor transient interaction between Rab6a(Q72L) and dynein in vivo using dual-colour fluorescence cross-correlation spectroscopy in dorsal root ganglion (DRG) neurons. Finally, we demonstrate that Rab6a(Q72L) mediates LIS1 release from a LIS1–dynein complex followed by dynein activation through an in vitro single-molecule assay using triple-colour quantum dots. Our findings reveal a surprising function for GTP bound Rab6a as an activator of idling dynein. Lissencephaly is a severe human neuronal migration defect characterized by a smooth cerebral surface, mental retardation and seizures [1] . The LIS1 gene was the first gene cloned in any organism important for neuronal migration, as it was deleted or mutated in humans with lissencephaly in a heterozygous manner [2] . LIS1 encodes a protein carrying seven WD (tryptophan-aspartate)-repeats [2] that was first identified as a non-catalytic subunit of platelet-activating factor acetylhydrolase 1b1 (ref. 3 ). LIS1 is a highly evolutionarily conserved protein that also includes NudF [4] in Aspergillus nidulans , Pac1 in Saccharomyces cerevisiae [5] and Dlis1 in Drosophila melanogaster [6] . In all of the organisms where they have been examined, LIS1 orthologues are complexed with cytoplasmic dynein, the main cytoplasmic microtubule (MT) ‘minus’-end-directed motor. Numerous studies to address the molecular function of LIS1 led to the conclusion that LIS1 is essential for the proper regulation and localization of cytoplasmic dynein [7] , [8] , [9] . We previously reported that LIS1 is essential for anterograde transport of cytoplasmic dynein in a kinesin-1-dependent manner and that mammalian nuclear distribution protein C (mNUDC) mediates the interaction between the LIS1–dynein complex and kinesin-1 (refs 9 , 10 ). We also reported that LIS1 and its binding protein, NDEL1, cooperatively regulate the plus-end-directed transport of cytoplasmic dynein. In addition, NDEL1 regulates MT organization with Aurora-A, which is essential for neurite extension [11] . Dynactin was first identified as a cytosolic activity that allowed cytoplasmic dynein to drive long-range movements of membrane vesicles on MTs in vitro [12] . Further work attributed the dynein-activating activity to a multiprotein complex [13] . Although mNUDC is required for anterograde transport of a dynactin-containing complex, the dynein complex and the dynactin complex were separately transported to the plus end of MTs [9] . Interestingly, half of the LIS1 is degraded through calpain-dependent proteolysis at the plus end of MTs, and that inhibition or knockdown of calpains protects LIS1 from proteolysis, which leads to the rescue of the phenotypes in Lis1 +/− mice [14] . Despite numerous studies for the regulation of motor proteins, the mechanism of LIS1 release from idling dynein at the plus end of MTs remains poorly understood. The process is essential to reactivate dynein motor in a retrograde fashion. A major retrograde route from the Golgi apparatus towards the endoplasmic reticulum (ER) involves vesicular coat complex coatomer protein I (COPI)-mediated transport [15] , [16] . Recent reports indicate the existence of a COPI-independent Golgi–ER retrograde pathway that functions as a recycling route for Golgi-resident glycosylation enzymes [17] , [18] , [19] . The COPI-independent pathway is regulated by the small GTPase Rab6a [18] , [20] . The dynein–dynactin-binding protein Bicaudal D1 and D2 colocalize with Rab6a on the trans -Golgi network (TGN) and cytoplasmic vesicles, and associate with Golgi membranes in a Rab6-dependent manner, suggesting that coordinated action between Rab6a, Bicaudal D and the dynein–dynactin complex controls COPI-independent Golgi–ER transport [21] . Here we show that Rab6a mediates LIS1 release from a LIS1–dynein complex followed by dynein activation. Our findings provide new insight into the role of guanosine triphosphate (GTP)-bound Rab6a as an activator of idling dynein. Rab6a dissociates LIS1 from a dynein idling complex We previously demonstrated that LIS1 arrests dynein motility ( Fig. 1a : lanes 1 and 2, Supplementary Movies 1 and 2 ) and that kinesin-1 transports a LIS1–dynein–tubulin complex to plus ends of MTs via mNUDC [9] , [10] . Before dynein can function as a retrograde motor, idling dynein must be activated to bind cargoes. It is currently believed that the bulk of dynactin participates in interactions with a wide range of cellular structures, many of which are cargoes of the dynein motor [22] . Therefore, we first examined whether a dynactin complex is able to release LIS1 from idling dynein and to activate dynein motility. A gliding assay revealed that a dynactin complex is able to partially activate dynein from an idling state ( Fig. 1a , Supplementary Movie 3 ). Five to ten minutes after application of dynactin, idling dynein fluctuated, but was not fully active ( Fig. 1a : lane 7). Bicaudal D is another multi-purpose adaptor of dynein. Bicaudal D and its highly similar mammalian homologues, Bicaudal D1 and D2, have been best characterized for their involvement in the dynein-mediated localization of mRNA throughout D. melanogaster development [23] and in the transport of Golgi vesicles in mammalian cells [24] . We next examined whether Bicaudal D is able to activate dynein by the gliding assay. Mouse Bicaudal D1 mildly augmented dynactin-mediated dynein activation, but activation was also incomplete ( Supplementary Movie 4 ). The small GTPase Rab6a is involved in the regulation of membrane traffic from the Golgi apparatus towards the ER in a COPI-independent pathway [17] , [18] , [20] . Bicaudal D1 and dynein light chain protein DYNLRB1 also colocalize with Rab6a on the TGN and cytoplasmic vesicles, and associate with Golgi membranes in a Rab6a-dependent manner [21] , [25] . Therefore, we investigated whether Rab6a modulates dynein activation. To our surprise, application of a constitutively active GTPase-deficient Rab6a mutant, Rab6a(Q72L) [21] , immediately and completely activated idling dynein and allowed it to resume MT transport, which was no obvious difference from dynein by itself ( Fig. 1a : lane 3, Supplementary Movie 5 ). In clear contrast, a guanosine diphosphate (GDP)-bound Rab6a mutant, Rab6a(T27N) [21] , did not display any activating properties ( Fig. 1a : lane 4, Supplementary Movie 6 ). Wild-type Rab6a-GTP displayed an intermediate function ( Fig. 1a : lane 5), whereas wild-type Rab6a-GDP did not display any activating functions ( Fig. 1a : lane 6). 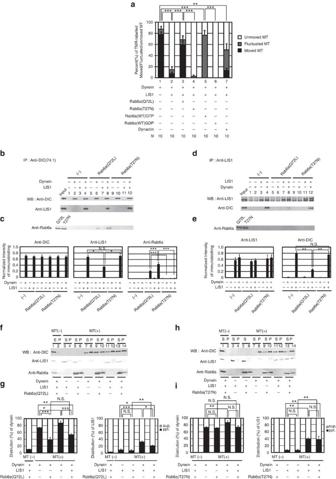Figure 1: Release of LIS1 from a LIS1–dynein complex and activation of dynein motility by GTP-bound form of Rab6a. (a) Summary of MT-gliding assay: percent of TMR-labelled MTs that displayed fluctuation (grey column) or gliding (black column). We used cytoplasmic dynein purified from porcine brain, which displayed approximately 0.5 μm s−1average gliding velocity. Conditions are shown at the bottom of the graph.N: observed number of chambers.P-values were calculated using a Student’st-test. (b) Immunoprecipitation assay using an anti-DIC antibody: protein combinations are shown at the top of the panels, and antibodies employed for western blotting (WB) are shown at the left side of the panels. (c) Quantitation of immunoprecipitation: precipitated DIC (left panel,N=3), LIS1 (middle panel,N=3) and Rab6a mutants (right panel,N=3), respectively, are shown. Each input for immunoblotting was expressed as 1.0.P-values were calculated using analysis of variance (ANOVA). (d) Immunoprecipitation assay using an anti-LIS1 antibody: applied protein combinations are shown at the top of the panels, and antibodies employed for WB are shown at the left side of the panels. (e) Quantitation of immunoprecipitation: precipitated LIS1 (left panel,N=3) and DIC (right panel,N=3) are shown. Each input for immunoblotting was expressed as 1.0.P-values were calculated using ANOVA. (f) MT pull-down assay using purified dynein, recombinant LIS1 and Rab6a(Q72L): protein combinations are shown at the bottom of the panels, and antibodies employed for WB are shown at the left side of the panels. (g) Quantitation of MT pull-down assay: co-precipitated dynein (left panel,N=6) and LIS1 (right panel,N=6) are shown.P-values were calculated using ANOVA. Note: Rab6a(Q72L) reduced dynein and LIS1, which were co-precipitated with MTs. (h) MT pull-down assay using dynein, LIS1 and Rab6a(T27N): protein combinations are shown at the bottom of the panels, and used antibodies for WB are shown at the left side of the panels. (i) Quantitation of MT pull-down assay: co-precipitated dynein (left panel,N=6) and LIS1 (right panel,N=6) are shown.P-values were calculated using ANOVA. All data expressed as mean±s.e.m. *P<0.05, **P<0.01 and ***P<0.001. N.S., not significant; ppt., precipitation; sup., supernatant. Figure 1: Release of LIS1 from a LIS1–dynein complex and activation of dynein motility by GTP-bound form of Rab6a. ( a ) Summary of MT-gliding assay: percent of TMR-labelled MTs that displayed fluctuation (grey column) or gliding (black column). We used cytoplasmic dynein purified from porcine brain, which displayed approximately 0.5 μm s −1 average gliding velocity. Conditions are shown at the bottom of the graph. N : observed number of chambers. P -values were calculated using a Student’s t -test. ( b ) Immunoprecipitation assay using an anti-DIC antibody: protein combinations are shown at the top of the panels, and antibodies employed for western blotting (WB) are shown at the left side of the panels. ( c ) Quantitation of immunoprecipitation: precipitated DIC (left panel, N =3), LIS1 (middle panel, N =3) and Rab6a mutants (right panel, N =3), respectively, are shown. Each input for immunoblotting was expressed as 1.0. P -values were calculated using analysis of variance (ANOVA). ( d ) Immunoprecipitation assay using an anti-LIS1 antibody: applied protein combinations are shown at the top of the panels, and antibodies employed for WB are shown at the left side of the panels. ( e ) Quantitation of immunoprecipitation: precipitated LIS1 (left panel, N =3) and DIC (right panel, N =3) are shown. Each input for immunoblotting was expressed as 1.0. P -values were calculated using ANOVA. ( f ) MT pull-down assay using purified dynein, recombinant LIS1 and Rab6a(Q72L): protein combinations are shown at the bottom of the panels, and antibodies employed for WB are shown at the left side of the panels. ( g ) Quantitation of MT pull-down assay: co-precipitated dynein (left panel, N =6) and LIS1 (right panel, N =6) are shown. P -values were calculated using ANOVA. Note: Rab6a(Q72L) reduced dynein and LIS1, which were co-precipitated with MTs. ( h ) MT pull-down assay using dynein, LIS1 and Rab6a(T27N): protein combinations are shown at the bottom of the panels, and used antibodies for WB are shown at the left side of the panels. ( i ) Quantitation of MT pull-down assay: co-precipitated dynein (left panel, N =6) and LIS1 (right panel, N =6) are shown. P -values were calculated using ANOVA. All data expressed as mean±s.e.m. * P <0.05, ** P <0.01 and *** P <0.001. N.S., not significant; ppt., precipitation; sup., supernatant. Full size image We next examined the effects of Rab6a on the interaction of LIS1 and dynein. First, we performed immunoprecipitation assays using purified dynein and LIS1 recombinant protein. Using an anti-dynein intermediate chain (DIC) antibody, we precipitated dynein complexes. LIS1 co-precipitated with dynein ( Fig. 1b : lane 4, Fig. 1c : middle panel). Rab6a(Q72L) also co-precipitated with dynein ( Fig. 1b : lane 6, Fig. 1c : right panel), indicating that Rab6a(Q72L) is able to bind dynein directly. Importantly, the amount of LIS1 co-precipitation was significantly reduced in the presence of Rab6a(Q72L) ( Fig. 1b : lane 8, Fig. 1c : middle panel), suggesting that Rab6a(Q72L) releases LIS1 from a LIS1–dynein complex. In contrast, Rab6a(T27N) was not able to bind dynein ( Fig. 1b : lane 10, Fig. 1c : right panel), and did not facilitate LIS1 dissociation ( Fig. 1b : lane 12, Fig. 1c : middle panel). We next reversed the combination. Using an anti-LIS1 antibody, we precipitated LIS1. Dynein co-precipitated with LIS1 ( Fig. 1d : lane 4). On the other hand, either nucleotide-bound form of Rab6a was not co-precipitated with LIS1 ( Fig. 1d : lanes 7, 8, 11 and 12), suggesting that Rab6a does not bind LIS1 directly. Rab6a(Q72L) reduced the amount of dynein that was co-precipitated with LIS1, but Rab6a(T27N) did not ( Fig. 1d : lanes 8 and 12, Fig. 1e : right panel). Next, we performed MT pull-down assay to examine the effects of Rab6a(Q72L) on dynein binding to MTs. Without MTs, the majority of dynein was distributed in the supernatant fraction, whereas the presence of MTs shifted dynein to the pellet fraction ( Fig. 1f : lanes 1, 2, 7 and 8, Fig. 1g : left). LIS1 augmented the proportion of dynein that was distributed in the pellet fraction ( Fig. 1f : lanes 11 and 12, Fig. 1g : left) [9] . Interestingly, Rab6a(Q72L) reduced the proportion of dynein that was distributed within the pellet fraction ( Fig. 1f : lanes 9 and 10, Fig. 1g : left). Importantly, Rab6a(Q72L) also reduced the proportion of dynein that was distributed within the pellet fraction in the presence of LIS1 ( Fig. 1f : lanes 13 and 14, Fig. 1g : left), suggesting that Rab6a(Q72L) erased the effect of LIS1 on dynein. In addition, Rab6a(Q72L) augmented the proportion of LIS1 that was distributed within the supernatant fraction ( Fig. 1f : lanes 11–14, Fig. 1g : right). In clear contrast, Rab6a(T27N) did not display such effects ( Fig. 1h ). Thus, we concluded that Rab6a(Q72L) expels LIS1 from a LIS1–dynein complex, to allow the activation of the dynein motor for retrograde movement. Interaction between dynein and Rab6a(Q72L) in DRG neurons Fluorescence correlation spectroscopy (FCS) can be used to attain additional information about molecular interactions in vivo . With FCS, the mobility of single-fluorescent molecules is detected by analysing the fluorescence fluctuations generated as individual molecule diffuse into and out of typical confocal detection volumes. The development of dual-colour fluorescence cross-correlation spectroscopy (FCCS) is a useful physical technique to determine molecular interaction quantitatively [26] , [27] , [28] . The method is also based on the temporal analysis of fluorescent amplitude fluctuations; if these fluctuations occur simultaneously in two channels, the proteins may be moving together in a complex. We therefore applied FCCS to examine whether dynein and Rab6a-GTP are cis -interacting in DRG neurons from postnatal mice. In the DRG neurons, each MT within the array is particularly oriented with its assembly-favoured plus end directed away from the cell body [9] . First, we examined the subcelluar localization of Rab6a by immunocytochemistry using a specific antibody and expressing enhanced green fluorescent protein (EGFP)-Rab6a in the DRG neurons. Interestingly, Rab6a accumulated at the plus ends close to the growth tip ( Supplementary Fig. S1a ). The Rab6a enriched region partially overlapped with the distribution of LIS1 ( Supplementary Fig. S1b ), suggesting that they may be localized at a potential dynein-loading zone [29] . We assumed that dynamic regulation for dynein loading was carried out within this loading zone, and focused FCCS examination onto the loading zone in the DRG neurons. For a negative control, we measured the cross-correlation for the interaction between EGFP and tetramethylrhodamine (TMR)-HaloTag fluorescent molecules using an EGFP and a TMR-HaloTag control vector ( Fig. 2a , Supplementary Fig. S3a ). We considered the cross-correlation for the negative control measurement as the background (relative cross amplitude (RCA)=0.028±0.024, mean±s.d.). Next, we examined the cross-correlation of EGFP-DIC1 and TMR-HaloTag-Rab6a (T27N), and found low levels of cross-correlation with the negative control (RCA=0.029±0.023, mean±s.d.) ( Fig. 2b ), which is consistent with low affinity binding between Rab6a (T27N) and dynein ( Fig. 1b , Supplementary Fig. S3b ). Importantly, TMR-HaloTag-Rab6a(Q72L) significantly augmented the cross-correlation (RCA=0.051±0.042, mean±s.d.) ( Fig. 2c , Supplementary Fig. S3c ). Subcellular distributions of TMR-HaloTag-Rab6a(T27N) and TMR-HaloTag-Rab6a(Q72L) did not display obvious differences ( Supplementary Fig. S2 ). We also examined the cross-correlation of EGFP-DIC1 and TMR-HaloTag-LIS1, and found a high level of cross-correlation between them (RCA=0.060±0.049, mean±s.d.) ( Fig. 2d , Supplementary Fig. S3d ). The series of FCCS analysis indicate that Rab6a(Q72L) interacts with dynein at the plus end of MTs in the vicinity of neurite tips in vivo . 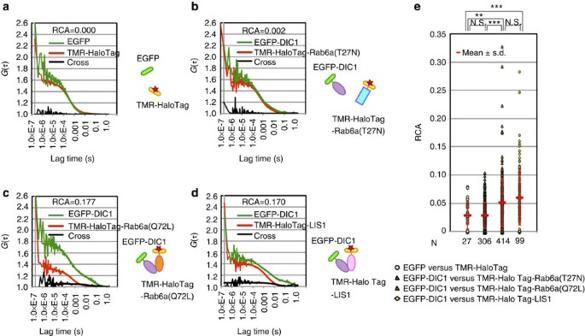Figure 2: Quantitation ofcis-interaction between dynein and Rab6a(Q72L) by FCCS at the periphery of DRG neurons. The inset is a schematic diagram demonstrating fluorescent-labelled proteins used with each experiment. Auto- and cross-correlation curves of fluorescent-labelled proteins were shown for EGFP and TMR-HaloTag (a), EGFP-DIC1 and TMR-HaloTag-Rab6a(T27N) (b), EGFP-DIC1 and TMR-HaloTag-Rab6a(Q72L) (c), and EGFP-DIC1 and TMR-HaloTag-LIS1 (d). (e) Statistics of FCCS data: the values of RCA were calculated and plotted.P-values were calculated using analysis of variance (**P<0.01, ***P<0.001). All data were expressed as mean±s.d. N.S., not significant. Figure 2: Quantitation of cis -interaction between dynein and Rab6a(Q72L) by FCCS at the periphery of DRG neurons. The inset is a schematic diagram demonstrating fluorescent-labelled proteins used with each experiment. Auto- and cross-correlation curves of fluorescent-labelled proteins were shown for EGFP and TMR-HaloTag ( a ), EGFP-DIC1 and TMR-HaloTag-Rab6a(T27N) ( b ), EGFP-DIC1 and TMR-HaloTag-Rab6a(Q72L) ( c ), and EGFP-DIC1 and TMR-HaloTag-LIS1 ( d ). ( e ) Statistics of FCCS data: the values of RCA were calculated and plotted. P -values were calculated using analysis of variance (** P <0.01, *** P <0.001). All data were expressed as mean±s.d. N.S., not significant. Full size image Co-migration of dynein and Rab6a(Q72L) in DRG neurons Although FCCS analysis demonstrated in vivo cis-interaction of dynein and Rab6a(Q72L), the direction of the movement cannot be defined. We applied total internal reflection fluorescence (TIRF) microscopy to trace the dynamics of dynein, Rab6a(Q72L) and LIS1, and determined the direction of their movement on MTs. TMR-HaloTag-Rab6a(Q72L) co-migrated with EGFP-DIC1 in DRG neurons ( Fig. 3a : left panel, Supplementary Movie 7 ). Importantly, they moved towards the soma without exception. We focused on this motile population and analysed the mean square displacement (MSD) of single-particle traces as a function of the time lagΔ t (that is, the difference between two time points) [30] . The MSDs were plotted and fitted by two equations, ρ (Δ t )=2 D Δ t + v 2 Δ t 2 –(1) and ρ (Δ t )=4 D Δ t + ζ –(2), where D is the diffusion coefficient, v is the (mean) velocity and ζ is noise term. If the particles of TMR-HaloTag-Rab6a(Q72L) or EGFP-DIC1 move in a directed constant-velocity fashion, that is, a purely ballistic scaling behaviour, the MSD would be fitted by equation (1), whereas if they move in purely random uncorrelated fashion, the MSD would be fitted by equation (2). Fitting analysis revealed that the MSDs of TMR-HaloTag-Rab6a(Q72L) and EGFP-DIC1 clearly fitted to Δ t 2 , suggesting that they behaved in a purely ballistic scaling manner, and were moving to the minus end of MTs (mean velocity±s.d. ( N =8), EGFP-DIC1: 0.54±0.26 μm s −1 , TMR-HaloTag-Rab6a(Q72L): 0.50±0.19 μm s −1 ) ( Fig. 3a : left panel, Table 1 , Supplementary Movie 7 ). In contrast, TMR-HaloTag-Rab6a(T27N) never displayed obvious co-migration with EGFP-DIC1 ( Fig. 3a : middle panel). However, EGFP-DIC1 by itself displayed ballistic scaling behaviour (mean velocity±s.d. ( N =10), TMR-HaloTag-Rab6a(T27N): 0.52±0.33 μm s −1 ) ( Fig. 3b : second panel from the left, Table 1 ). Finally, EGFP-DIC1 and TMR-HaloTag-LIS1 displayed co-migration to the tip of neurite processes (mean velocity±s.d. ( N =10), EGFP-DIC1: 0.47±0.27 μm s −1 , TMR-HaloTag-LIS1: 0.43±0.24 μm s −1 ), suggesting that they are moving to the plus end of MTs as we demonstrated previouly [9] ( Fig. 3a : right panel, Table 1 ). The MSDs of EGFP-DIC1 and TMR-HaloTag-LIS1 also fitted to Δ t 2 , suggesting that they were behaving as ballistic scaling ( Fig. 3b : right two panels, Supplementary Movie 8 ). Thus, we concluded that dynein directly binds to an active form of Rab6a, but not to an inactive form, and moves in the minus-end direction of MTs. We assume that activation of Rab6a releases LIS1 from a dynein idling complex and triggers retrograde movement. 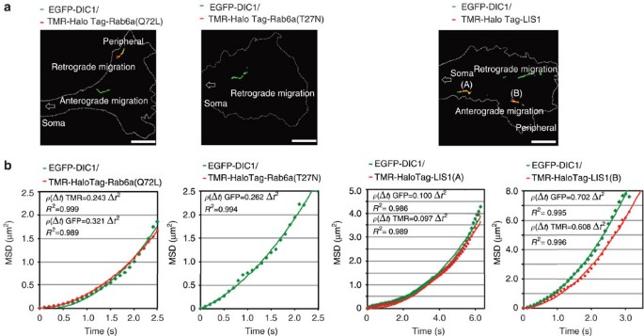Figure 3: Demonstration of co-migration of dynein and Rab6a(Q72L) at the periphery of DRG neurons by TIRF. (a) Representative traces in the DRG neuorns by TIRF microscopy expressed with: EGFP-DIC1 and TMR-HaloTag-Rab6a(Q72L) (left panel), EGFP-DIC1 and TMR-HaloTag-Rab6a(T27N) (middle panel), and EGFP-DIC1 and TMR-HaloTag-LIS1 (right panels). White arrows indicate the direction towards the soma. The direction of transport was defined by the orientation of transport. Note: TMR-HaloTag-Rab6a(Q72L) co-migrated with EGFP-DIC1 in a retrograde fashion, whereas TMR-HaloTag-LIS1 co-migrated with EGFP-DIC1 in an anterograde fashion. TMR-HaloTag-Rab6a(T27N) did not display obvious co-migration. Scale bar, 5 μm. (b) MSDs were calculated from the motility of: EGFP-DIC1 and TMR-HaloTag-Rab6a(Q72L) (left panel); EGFP-DIC1 (second panel from the left); and EGFP-DIC1 and TMR-HaloTag-LIS1 (right two panels). Fits represent MSDρ(Δt)=2DΔt+ν2Δt2.Note:traces of EGFP-DIC1, TMR-HaloTag-Rab6a(Q72L) and TMR-HaloTag-LIS1 fit second-order polynomial MSD (Δt), indicating that they are following ballistic scaling behaviour, rather than diffusive scaling behaviour. Figure 3: Demonstration of co-migration of dynein and Rab6a(Q72L) at the periphery of DRG neurons by TIRF. ( a ) Representative traces in the DRG neuorns by TIRF microscopy expressed with: EGFP-DIC1 and TMR-HaloTag-Rab6a(Q72L) (left panel), EGFP-DIC1 and TMR-HaloTag-Rab6a(T27N) (middle panel), and EGFP-DIC1 and TMR-HaloTag-LIS1 (right panels). White arrows indicate the direction towards the soma. The direction of transport was defined by the orientation of transport. Note: TMR-HaloTag-Rab6a(Q72L) co-migrated with EGFP-DIC1 in a retrograde fashion, whereas TMR-HaloTag-LIS1 co-migrated with EGFP-DIC1 in an anterograde fashion. TMR-HaloTag-Rab6a(T27N) did not display obvious co-migration. Scale bar, 5 μm. ( b ) MSDs were calculated from the motility of: EGFP-DIC1 and TMR-HaloTag-Rab6a(Q72L) (left panel); EGFP-DIC1 (second panel from the left); and EGFP-DIC1 and TMR-HaloTag-LIS1 (right two panels). Fits represent MSD ρ (Δ t )=2 D Δ t + ν 2 Δ t 2 . Note: traces of EGFP-DIC1, TMR-HaloTag-Rab6a(Q72L) and TMR-HaloTag-LIS1 fit second-order polynomial MSD (Δ t ), indicating that they are following ballistic scaling behaviour, rather than diffusive scaling behaviour. Full size image Table 1 Summary table of the mean velocity, calculated by each MSD curve. Full size table Rab6a(Q72L) releases LIS1 and activates dynein motility Finally, we performed in vitro single-molecule assays using purified dynein, as well as recombinant proteins of Rab6a and LIS1 to confirm our model. To be able to accurately follow single-dynein dimers during their entire runs along MTs that were adsorbed onto the surface of a microscope perfusion chamber, we used Q-dots as extremely photostable fluorescent probes. This eliminated the problem of photobleaching that might obscure part of the run. Dynein was linked to 605 nm Q-dot using an antibody (clone: 74.1) to the intermediate chain, which was covalently bound to the surface of 605 nm Q-dot by a 1-ethyl-3-(3-dimethylaminopropyl) carbodiimide coupling reaction. LIS1 and Rab6a(Q72L) were conjugated to 525 nm Q-dot and 655 nm Q-dots via a SNAP-tag that was attached to the N-terminus, respectively. Kymographs of dynein (spatiotemporal plots) demonstrated that individual runs had roughly constant velocities ( Supplementary Fig. S4a,b , Supplementary Movie 9 ). In agreement with single-molecule studies of dynein labelled with fluorophores [31] , the velocities measured for many individual runs displayed a Gaussian distribution with a mean velocity of 0.53±0.05 μm s −1 (mean±s.d., N =121) ( Supplementary Fig. S4c ), and the run lengths of the individual runs demonstrated an exponential distribution with an overall average run length of 1.57±0.44 μm (mean±s.d., N =165) ( Supplementary Fig. S4d ) [31] . We next confirmed LIS1-mediated suppression of dynein motility ( Supplementary Fig. S4e,f , Supplementary Movie 10 ). Although our in vitro single-molecule assays indicate that LIS1 inhibits dynein motility, it might be possible that LIS1-bound dynein is still mobile within the small level, in which the spatial resolution of our method cannot dissect [32] . Using this system, we examined whether Rab6a is able to release LIS1 from the LIS1–dynein complex and to activate dynein motility. First, we examined the coexistence of LIS1 and dynein on MTs, and found that LIS1 and dynein clearly coexisted stably on MTs ( Supplementary Fig. S4h ), which were still detectable 10 min after the administration of control buffer ( Supplementary Fig. S4h , left panel). In contrast, the addition of the unconjugated form of Rab6a(Q72L) released LIS1 from LIS1–dynein complexes and resulted in the gradual disappearance of dynein on MTs 10 min after administration of Rab6a(Q72L) ( Supplementary Fig. S4h , right panel). By contrast, administration of Rab6a(T27N) did not result in obvious effects on the LIS1–dynein complexes, which exhibited a similar pattern as controls ( Supplementary Fig. S4h , left and middle panels). These observations suggest that Rab6a(Q72L) is able to displace LIS1 from LIS1–dynein complexes and to activate dynein motility, but Rab6a(T27N) is not, consistent with our previous results. Next, we wanted to address whether Rab6a(Q72L) can displace LIS1 from LIS1–dynein complexes and to activate dynein motility using triple-colour Q-dots. Dynein and LIS1 together resulted in an immobile complex on MTs ( Supplementary Fig. S4e,g , Supplementary Movie 10 ). Rab6a(Q72L) approached this complex and made a transient triple complex, which was followed by the immediate dissociation of LIS1 resulting in a mobile dynein–Rab6a(Q72L) complex ( Fig. 4a , Supplementary Movie 11 , Supplementary Fig. S4i ). We next tracked individual Q-dots of dynein and Rab6a(Q72L), which revealed co-migration with a velocity of approximately 0.47±0.15 μm s −1 (mean±s.d. ), suggesting that dynein and Rab6a(Q72L) made a complex ( Fig. 4 ). Rab6a(Q72L)-mediated LIS1 dissociation is a very rapid reaction, one that is significantly shorter than the average binding duration of the LIS1–dynein complex (33–50 s, Supplementary Fig. S4g ). We interpret these findings to demonstrate that Rab6a(Q72L) actively releases, rather than spontaneously dissociates, LIS1 from the dynein complex. A recent study reported that both dynein and its cargo moved at normal speeds in the absence of LIS1, and that LIS1, unlike dynein and dynactin, was absent from moving dynein cargos, further suggesting that LIS1 is not required for dynein-based cargo motility once it has commenced [33] . 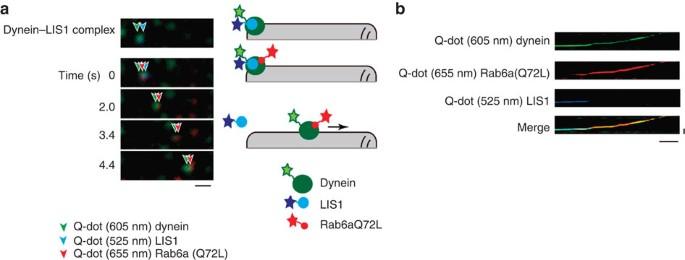Figure 4: LIS1 release from a LIS–dynein complex by Rab6a(Q72L), and the activation of dynein motility on MTs. Single-molecule movement of dynein, LIS1 and Rab6a(Q72L) coupled to Q-dots. (a) TIRF microscopic images of Q-dot-conjugated 605 Q-dot dynein (λ(emission)=605 nm, green), 525 Q-dot LIS1 (λ(emission)=525 nm, blue) and 655 Q-dot Rab6a(Q72L) (λ(emission)=655, red) are shown. The green, blue and red arrowheads indicate dynein, LIS1 and Rab6a(Q72L), respectively. Schematic combinations are shown at the right side. Rab6a(Q72L) facilitated dissociation of LIS1 from the LIS1–dynein idling complex. Released LIS1 disappeared. Scale bar, 1.0 μm. (b) The kymograph patterns of dynein (green line), Rab6a(Q72L) (red line) and LIS1 (blue line) are shown. Vertical scale bar, 1.0 μm; Horizontal scale bar, 1.0 s. Figure 4: LIS1 release from a LIS–dynein complex by Rab6a(Q72L), and the activation of dynein motility on MTs. Single-molecule movement of dynein, LIS1 and Rab6a(Q72L) coupled to Q-dots. ( a ) TIRF microscopic images of Q-dot-conjugated 605 Q-dot dynein ( λ (emission)=605 nm, green), 525 Q-dot LIS1 ( λ (emission)=525 nm, blue) and 655 Q-dot Rab6a(Q72L) ( λ (emission)=655, red) are shown. The green, blue and red arrowheads indicate dynein, LIS1 and Rab6a(Q72L), respectively. Schematic combinations are shown at the right side. Rab6a(Q72L) facilitated dissociation of LIS1 from the LIS1–dynein idling complex. Released LIS1 disappeared. Scale bar, 1.0 μm. ( b ) The kymograph patterns of dynein (green line), Rab6a(Q72L) (red line) and LIS1 (blue line) are shown. Vertical scale bar, 1.0 μm; Horizontal scale bar, 1.0 s. Full size image The clear prediction from their model is that loss of Rab6a function should result in the failure to activate dynein at the plus end of MTs. To address this question, we performed small interfering RNA (siRNA)-mediated Rab6a-knockdown experiments. After depletion of Rab6a by siRNA, we found that aberrant accumulation of cytoplasmic dynein at the plus end of MTs, which is consistent with our model ( Fig. 5 , Supplementary Fig. S5 ). In addition, another report demonstrated that knocking down the expression of Rab6a hampers the intracellular transport of the retrograde cargo marker, the Shiga Toxin B subunit along the endocytic pathway [34] . Thus, we concluded that Rab6a-mediated dynein activation is critically important for cargo loading in vivo . 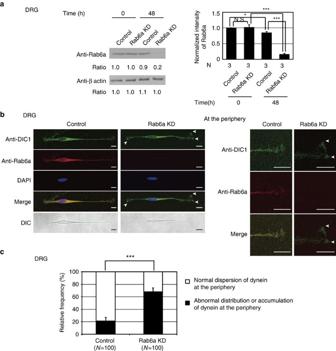Figure 5: Knockdown of Rab6a results in an abnormal localization of dynein at the periphery of the DRGs. Down regulation of Rab6a by siRNA in DRG cells. (a) Western blotting analysis of Rab6a 48 h (or 0 h) after transfection with siRNA-targeting mouse Rab6a or pGL2 (left panel). Quantitation of normalized immunoblot values (right panel).P-values were calculated using a Student’st-test (*P<0.05 and ***P<0.001). All data are expressed as mean±s.e.m. (b) Immunocytochemistry data 48 h after transfection with each of the siRNAs. Endogenous expression of Rab6a and DIC in the DRG neurons using the specific antibody for Rab6a and DIC. Note: Depletion of Rab6a induced an abnormal localization and accumulation of dynein at the periphery of the DRG cells. Scale bar, 10 μm. (c) Each percentage of aberrant distribution of dynein was presented, which was preferentially observed in Rab6a-depleted DRG neurons.Nindicates the number of examined DRG neurons with independent four experiments.P-values were calculated using a Student’st-test (***P<0.001). All data are expressed as mean±s.e.m. DAPI, 4',6-diamidino-2-phenylindole; N.S., not significant. Figure 5: Knockdown of Rab6a results in an abnormal localization of dynein at the periphery of the DRGs. Down regulation of Rab6a by siRNA in DRG cells. ( a ) Western blotting analysis of Rab6a 48 h (or 0 h) after transfection with siRNA-targeting mouse Rab6a or pGL2 (left panel). Quantitation of normalized immunoblot values (right panel). P -values were calculated using a Student’s t -test (* P <0.05 and *** P <0.001). All data are expressed as mean±s.e.m. ( b ) Immunocytochemistry data 48 h after transfection with each of the siRNAs. Endogenous expression of Rab6a and DIC in the DRG neurons using the specific antibody for Rab6a and DIC. Note: Depletion of Rab6a induced an abnormal localization and accumulation of dynein at the periphery of the DRG cells. Scale bar, 10 μm. ( c ) Each percentage of aberrant distribution of dynein was presented, which was preferentially observed in Rab6a-depleted DRG neurons. N indicates the number of examined DRG neurons with independent four experiments. P -values were calculated using a Student’s t -test (*** P <0.001). All data are expressed as mean±s.e.m. DAPI, 4',6-diamidino-2-phenylindole; N.S., not significant. Full size image In this paper, we demonstrated that idling dynein is a direct target of Rab6a. Rab6a releases LIS1 from the LIS1–dynein idling complex to allow the resumption of dynein motor activity. On the other hand, NDEL1s are also required for the activation of dynein that is bound with LIS1 as we reported previously [9] . In our present model, Rab6a adequately releases LIS1 from dynein, resulting in LIS1-free dynein molecules. Further investigation is needed to clarify the role of NDEL1 in the dynein activation. An interesting question is how does Rab6a release LIS1 from dynein? One possibility is that they are simply competing for the same binding position. Another possibility is that Rab6a might bind to a distinct position of dynein, which induce allosteric modification. Rab6a(Q72L) has significantly higher affinity for the LIS1–dynein complex, suggesting that the molecular mechanism of Rab6a(Q72L)-mediated LIS1 dissociation might not be attributable to simple competition. The LIS1-binding position on dynein was recently determined [32] . Rab6a might induce a structural modification, resulting in decreased LIS1-binding affinity. Rab proteins were identified as potent regulatory molecules of motor protein recruitment. Members of the Rab family are specifically targeted to intracellular vesicles and organelles, where they serve as molecular switches as they cycle between GTP-bound and GDP-bound forms, which each recruit a different set of effectors [35] , [36] , [37] . Rabs also recruit molecular motors and therefore regulate transport between donor and acceptor compartments, including the recruitment of a kinesin to endosomes [38] and the recruitment of dynein to the TGN [21] , [39] . In particularly, Rab6a binds to dynactin [39] , a protein that binds dynein directly and allows the motor to traverse the MT lattice over long distances. Dynactin is also required for the binding of membrane vesicles with dynein [22] . Presumably, Rab6a mediates sequential reactions, in which Rab6a releases LIS1 to activate the dynein motor as well as facilitate cargo loading on the dynein motor, ensuring the efficient creation of the cargo–dynein transport complex from the LIS1–dynein idling complex. Currently, over 60 small GTPase Rab family proteins are recognized. Among them, other Rabs may be present for activation of dynein in a similar fashion. Rab proteins are further regulated by a diverse group of structurally unrelated GDP–GTP exchange factors and a family of GTP-hydrolysis-activating proteins [40] , [41] . For example, various DENN domains interact directly with members of the Rab family of small GTPases, and DENN (differentially expressed in normal and neoplastic cells) domains function enzymatically as Rab-specific guanine nucleotide exchange factors [42] , [43] . There are 18 genes encoding DENN domain-containing proteins in humans [44] . Therefore, it is possible to create numerous combinations of Rabs and its regulatory proteins including GTP-hydrolysis-activating proteins and GDP–GTP exchange factors, to adapt the fine regulation of complicated intracellular transport that is driven by the dynein motor. Vectors used for expression in DRG and recombinant proteins Complementary DNAs carrying full-length open-reading frames of each of the proteins were conjugated to pEGFP (Clonetech Laboratories, CA, USA) or HaloTag vectors (Promega, WI, USA). The TMR (Promega) ligand was used for HaloTag detection. Recombinant proteins for LIS1 and each of Rab6a’s (wild-type, Q72L and T27N) were generated using baculovirus-insect cell expression system (Invitrogen) and pGEX-4T expression vector (GE Healthcare Lifesciences, UK), respectively. Recombinant proteins were purified as described in Supplementary Methods . DRG preparation and cell culture DRG preparation was performed as described in Supplementary Methods . The DRGs were transfected with vectors to express various proteins immediately after dissection using the Neon transfection system (Life Technologies, CA, USA) [3] . The cells were plated onto poly- D -lysine-coated dishes (MatTek, MA, USA) and cultured in DMEM (Wako Chemicals, Osaka, Japan) with 10% heat-inactivated fetal bovine serum (Nichirei Biosciences, Tokyo, Japan), 200 ng ml −1 2.5S mNGF (Sigma-Aldrich, MO, USA) and 5 μM uridine/deoxyfluorouridine (Sigma-Aldrich) for 48 h. Small interfering RNA The targeted sequence of mouse Rab6a: 5′-GUUGGAAAGACGUCCUUGATT-3′ and a firefly ( Photinus pyralis ) luciferase (pGL2): 5′-CGUACGCGGAAUACUUCGATT-3′ as a negative control were synthesized by Sigma-Aldrich. Each double-stranded 21-nucleotide RNA at a final concentration of 200 nM was transfected into the DRGs using the Neon transfection system (Life Technologies). FCS and FCCS measurements FCS and FCCS measurements were performed on an LSM 710META confocal laser scanning microscope plus ConfoCor3 system (Carl Zeiss, Oberkochen, Germany). Argon-ion (488 nm) and Helium–Neon (543 nm) lasers were simultaneously focused through a C-Apochromat × 40, numerical aperture (NA) 1.2, water objective lens (Carl Zeiss). The laser power for the Argon-ion and Helium–Neon lasers were within the range of 2.0–8.3 and 3.7–6.0 μW, respectively. This power level is high enough to observe the fluorescence signal from each molecule and still low enough to maintain low levels of photobleaching. The confocal pinhole diameters were adjusted to 32 μm. The emission signals were split through a dichroic mirror (600 nm beam splitter) and detected with a band-pass filter (505–530 nm) and a long-pass filter (615–680 nm) for green and red fluorescence, respectively. The confocal detection volume was ~0.23 fl. Data were acquired in 5 s × 10 times per a region. All measurements were performed at 37 °C. In FCS measurements, fluctuation δI ( t ) in the detected fluorescence intensity I ( t ) is typically generated as molecule diffuse in and out of a focused laser beam. An auto-correlation function G ( τ ) was calculated from fluctuations of the fluorescence intensity as follows: τ is a lag time for correlation function. G gr( τ ) denotes a cross-correlation function calculated from fluctuations δ I g( t ) and δ I r( t ) of the fluorescence intensity in green (g), red (r) and overlapping (gr) volume as follows: I g( t ) and I r( t ) are time-dependent fluorescence intensity in the green channel or the red channel, respectively. Auto- and cross-correlation curves obtained from FCS and FCCS measurements allow the determination of the particle number and the diffusion time of single-colour molecules, as well as the particle number of dual-colour molecules, respectively [45] . The average numbers of green fluorescent particles ( N g ), red fluorescent particles ( N r ), and particles that have both red and green fluorescence ( N gr ) in the confocal volume can be calculated by: For interaction studies between two species labelled with EGFP (g) and TMR-HaloTag (r), RCA was defined as follows: Equation (5) follows from equations (3) and (4): In vivo single-molecule fluorescence imaging Fluorescence images were obtained using an inverted microscope (TE2000-U; Nikon Instech, Tokyo, Japan) through an oil immersion objective lens (PlanApo × 100, NA 1.49, Nikon Instech). Both EGFP-DIC1 and TMR-labelled HaloTag-Rab6a mutants Q72L, T27N or LIS1 were excited simultaneously by a 488-nm Argon-ion laser (532-BS-A04; Omnichrome, CA, USA). By using dual-view optics (A8509; Hamamatsu Photonics, Hamamatsu, Japan), each emission was split into two parts at 550 nm by a dichroic mirror (DM550LP and DM550SP; Hamamatsu Photonics). The split images were passed through an emission filter (FF01-525/45-25 for EGFP and FF01-593/40-25 for TMR; Semrock, IL, USA) and captured simultaneously by an electron multiplying CCD (charge-coupled device) camera (DU-897BV; Andor Technology, UK). All experiments were performed at 37 °C with a stage incubator (Tokai-Hit, Shizuoka, Japan). For the single-particle tracking of EGFP or TMR-HaloTag fusion proteins, the peripherals at the DRGs were continuously observed. Time-lapse images were acquired at 100-ms intervals and further processed using Image J software (National Institutes of Health, MD, USA) with self-work particle-tracking plugins developed by Y.A. To further analyse the movement of fluorescent-labelled molecule, the MSD ( ρ (Δ t )) against time, which is a convenient quantitative measure of stochastic movement, was calculated by Octave software. The MSD was plotted and fitted by two equations, ρ 2(Δ t )=2 D Δ t + ν 2 Δ t 2 and ρ 1(Δ t )=4 D Δ t + ζ , where D is the diffusion coefficient, ν is the (mean) velocity and ζ is noise term. In vitro MT-gliding assay In vitro MT-gliding assays were performed as described in Supplementary Methods . MT-binding assays Purified dynein from porcine brain was mixed with recombinant LIS1 in the absence or presence of recombinant Rab6a(Q72L) or Rab6a(T27N). The MAP-depleted tubulin (7.5 mg ml −1 ) was assembled in 50 μM taxol, then mixed with dynein at 62 μg ml −1 . Some of the samples were treated with LIS1 (0.4 μM) and/or each Rab6a mutant (0.8 μM). After incubation for 5 min at room temperature, MTs were collected by centrifugation at 200 000 g for 10 min at room temperature using a 120.2 rotor in an Optima TLX ultracentrifuge (Beckman Coulter, CA, USA). The supernatants and pellets were separated and subjected to electrophoresis. After electrophoresis, proteins were transferred to polyvinylidene difluoride membrane. The blots were probed with anti-Rab6 rabbit polyclonal antibody (1,000 × dilution) (Merck Millipore, MA, USA), anti-cytoplasmic DIC mouse monoclonal antibody (clone: 74.1) (1,000 × dilution) (Merck Millipore) and anti-LIS1 (1,000 × dilution), which we made, and the bands were digitized and quantified by LAS3000 (FUJI FILM, Tokyo, Japan). Immunoprecipitation and immunocytochemistry These methods were described in Supplementary Methods . In vitro single-molecule assay The previously described in vitro motility assay was modified for single-molecule assays using TIRF microscopy [3] . Tubulin purified from fresh porcine brain was labelled with TMR (FluoReporter TMR Protein Labelling Kit; Life Technologies) and polymerized in 25K-Ace buffer (25 mM CH 3 COOK, 4 mM MgSO 4 , 1 mM EGTA, 10 mM PIPES-KOH(pH 6.8) and 1 mM dithiothreitol) containing 1 mM GTP, and 33 μM Taxol was added to maintain MT polymerization. First, anti-α tubulin (2 × dilution) (TU-02; Santa Cruz Biotechnology) was introduced into the observation chamber and absorbed onto the glass for 5 min. The following were then added in sequence: (i) Blocking buffer (4 μg ml −1 of casein in 25K-Ace buffer to remove the unabsorbed antibody and block the glass surface for 2 min); ii) Taxol-stabilized MTs in blocking buffer containing 33 μM Taxol and an oxygen scavenger (10 mM glucose, 50 μg ml −1 glucose oxidase, 9 μg ml −1 catalase and 1% β-mercaptoethanol); (iii) Blocking buffer to remove the unabsorbed MT and further block the glass surface. For labelling, purified dynein with 605 Q-dot ( λ (emission)=605 nm; Life Technologies) was cross-linked to anti-DIC antibody (clone: 74.1; Merck Millipore, MA, USA) via 1-ethyl-3-(3-dimethylaminopropyl) carbodiimide (Fluka, Buchs, Switzerland), and then mixed with dynein. SNAP-tagged LIS1 and SNAP-tagged Rab6a(Q72L) were labelled with 525 Q-dot ( λ (emission)=525 nm; Life Technologies) and 655 Q-dot ( λ (emission)=655 nm; Life Technologies) using the SNAP-tag ligand (New England Biolabs, MA, USA), respectively. The 605 Q-dot dynein was introduced into the observation chamber. After incubation for 5 min, the chamber was rinsed by blocking buffer to remove excess 605 Q-dot dynein, and motility buffer (25K-Ace buffer supplemented with 1 mM ATP, 33 μM taxol, 1 mM dithiothreitol and 1 mM GTP) containing the oxygen scavenger system was applied. Single-fluorescent images of 605Q-dot dynein, 525Q-dot LIS1 and 655Q-dot Rab6a(Q72L) were obtained by a custom-built TIRF microscope through an oil immersion objective lens (ApoN × 60, NA 1.49, Olympus, Tokyo, Japan). 605 Q-dot dynein, 525 Q-dot LIS1 and 655 Q-dot Rab6a were excited simultaneously by a 488-nm laser at 100 mW (Sapphire; Coherent, CA, USA). The split images were passed through each emission filter (Brightline; Semrock) and captured simultaneously by an electron multiplying CCD camera (iXon; Andor Technology, Belfast, Northern Ireland). Time-lapse images were acquired at 33-ms intervals and further processed using ImageJ software (National Institutes of Health, MD, USA). We first fixed the Q-dot to the DIC antibody molar ratio was 1:1. To ensure that Q-dot movement on MTs was being driven by a single kinesin motor, we further varied the Q-dot to dynein molar ratio from 1:2 to 1:0.2, and examined run length. In all conditions, Q-dot-conjugated dynein displayed stable and the characteristic run length, which we concluded that majority of Q-dot bound to a single dynein. We finally applied the Q-dot to dynein molar ratio with 1:0.2 for further experiments. All experiments were performed at 37 °C with a stage incubator (Tokai-Hit). How to cite this article: Yamada, M. et al. Rab6a releases LIS1 from a dynein idling complex and activates dynein for retrograde movement. Nat. Commun. 4:2033 doi: 10.1038/ncomms3033 (2013).